Extreme binocular vision and a straight bill facilitate tool use in New Caledonian crows Humans are expert tool users, who manipulate objects with dextrous hands and precise visual control. Surprisingly, morphological predispositions, or adaptations, for tool use have rarely been examined in non-human animals. New Caledonian crows Corvus moneduloides use their bills to craft complex tools from sticks, leaves and other materials, before inserting them into deadwood or vegetation to extract prey. Here we show that tool use in these birds is facilitated by an unusual visual-field topography and bill shape. Their visual field has substantially greater binocular overlap than that of any other bird species investigated to date, including six non-tool-using corvids. Furthermore, their unusually straight bill enables a stable grip on tools, and raises the tool tip into their visual field's binocular sector. These features enable a degree of tool control that would be impossible in other corvids, despite their comparable cognitive abilities. To our knowledge, this is the first evidence for tool-use-related morphological features outside the hominin lineage. Tool-using animals must be able to hold tools firmly and guide them accurately. Humans possess several morphological features that aid their precise handling and deployment of tools, including a powerful visual system for accurate relative depth perception [1] , and hands with opposable thumbs for a secure grip [2] , [3] . Comparatively few non-human animal species are known to use tools in the wild [4] , and it remains unknown whether any of them benefit from similar morphological predispositions or adaptations. New Caledonian crows Corvus moneduloides ('NC crows' hereafter) use tools for extractive foraging [5] , exhibiting a remarkable degree of dexterity. Using their bills, these tropical birds craft complex tools from sticks, leaf edges and other materials, before inserting them into deadwood or vegetation to 'fish' for invertebrate prey [6] . In this study, we show that NC crows present at least two unusual morphological features that combine to facilitate their use of tools: extreme binocular vision and an uncharacteristically straight bill. Taken together, these adaptations enable a secure grip and accurate visual guidance of the tool, even when probing into narrow holes. 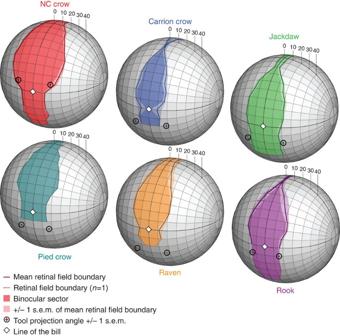Figure 1: Visual-field projections on orthographically viewed spheres for sixCorvusspecies. The diagrams use a conventional latitude and longitude coordinate system (with 10° intervals), aligned so that the bill tip is in line with the eyes in the horizontal plane, and the median sagittal plane of the skull (denoted by the white kite shapes). It should be imagined that the bird's head is positioned at the centre of the transparent sphere, with the bill tip and field boundaries projected onto the surface of the sphere. Estimated tool-projection angles are plotted onto the spheres, to examine to what degree the six different species can potentially rely on visual feedback of tool-tip position during tool deployment. Only in the NC crow do the tool-projection angles fall completely within the binocular sector, such that the contralateral eye is able to see along the tool (cf.Fig. 4). Visual-field topography We measured visual-field parameters (monocular, binocular and cyclopean fields) and eye-movement amplitudes in 18 alert subjects from 6 Corvus species ( Figs 1 and 2 and Table 1 ), using a well-established ophthalmoscopic reflex technique [7] . NC crows had a mean (±s.e.m.) maximum binocular overlap of 61.5°±0.2 ( n =3), which is much greater (by between 14.8° and 23.9°; see Table 1 ) than that observed in the five non-tool-using Corvus species examined in this study, and a previously reported value for American crows C. brachyrhynchos [8] . This striking degree of binocularity appears to be at least partly due to unusually large eye-movement amplitudes ( Table 1 ). The average maximum binocular field width of NC crows exceeded that of other Corvus species over 140° of elevation, spanning from the bill tip to behind the head ( Fig. 1 ). Figure 1: Visual-field projections on orthographically viewed spheres for six Corvus species. The diagrams use a conventional latitude and longitude coordinate system (with 10° intervals), aligned so that the bill tip is in line with the eyes in the horizontal plane, and the median sagittal plane of the skull (denoted by the white kite shapes). It should be imagined that the bird's head is positioned at the centre of the transparent sphere, with the bill tip and field boundaries projected onto the surface of the sphere. Estimated tool-projection angles are plotted onto the spheres, to examine to what degree the six different species can potentially rely on visual feedback of tool-tip position during tool deployment. Only in the NC crow do the tool-projection angles fall completely within the binocular sector, such that the contralateral eye is able to see along the tool ( cf. Fig. 4 ). 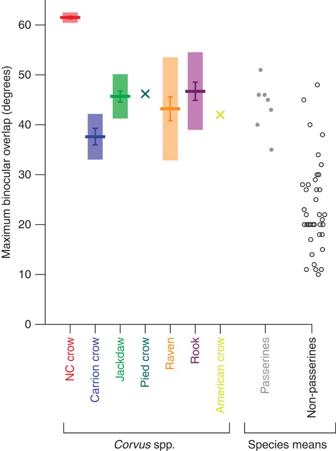Figure 2: Maximum binocular overlap in tool-using NC crows and non-tool-using control species. For theCorvusspecies, mean values are shown with s.e.m. (vertical bars) and 95% confidence intervals (shaded boxes), except for the pied crow (single data point) and the American crow (previously published mean value8); colour coding is the same as inFig. 1. For the samples of other passerine and non-passerine birds, datapoints are (horizontally jittered) species values (means where available; seeSupplementary Table S1). Although the degree of binocularity in non-tool-usingCorvusspecies is similar to that of all other passerines measured to date, NC crows represent a highly significant outlier in this sample (seeTable 1). Measurements for corvids were obtained as part of this study (except for the American crow), and all other data were collated through an exhaustive literature review (seeSupplementary Table S1). Full size image Figure 2: Maximum binocular overlap in tool-using NC crows and non-tool-using control species. For the Corvus species, mean values are shown with s.e.m. (vertical bars) and 95% confidence intervals (shaded boxes), except for the pied crow (single data point) and the American crow (previously published mean value [8] ); colour coding is the same as in Fig. 1 . For the samples of other passerine and non-passerine birds, datapoints are (horizontally jittered) species values (means where available; see Supplementary Table S1 ). Although the degree of binocularity in non-tool-using Corvus species is similar to that of all other passerines measured to date, NC crows represent a highly significant outlier in this sample (see Table 1 ). Measurements for corvids were obtained as part of this study (except for the American crow), and all other data were collated through an exhaustive literature review (see Supplementary Table S1 ). Full size image Table 1 ∣ Visual-field parameters for seven Corvus species and other birds. Full size table An exhaustive review of previously published material on avian visual fields yielded comparative data for 46 bird species across 19 orders ( Supplementary Table S1 ). NC crows exhibited considerably larger maximum binocular overlap than all other passerines ( Corvus species excluded) and all non-passerines in this database ( Fig. 2 , Table 1 , Supplementary Table S1 ), exceeding the highest species values by 10.5° and 13.5°, respectively. Visual control during tool deployment To examine the hypothesis that the unusual visual-field topography of NC crows supports their tool-use behaviour, we conducted behavioural experiments with three wild-caught subjects. Using a custom-built infrared ophthalmoscope video camera hidden at the base of a baited tube (which mimicked the shape of natural foraging holes), we filmed the crows' eye movements and tool handling during unconstrained tool use (Methods). Our video analyses revealed that NC crows bring both eyes forward during tool use, maximising the contralateral projections of each eye's visual field ( Fig. 3 ). During stick-tool use, NC crows typically hold the tool in their bill tip, with the non-working end of the tool either held against one cheek ('angled' grip; Fig. 4a, and position 1 in Fig. 4b ) or inside the bill ('straight' grip; position 2 in Fig. 4b ) [9] , [10] . We found that, when the aperture of the experimental hole was large enough for both eyes to see into, our subjects strongly preferred an angled grip over a straight grip (generalized linear mixed model (GLMM), comparison between large and small aperture: n =118 trials, 3 individuals, z =−6.78, P <0.001). In this configuration, the species' extensive binocular overlap enables a bird to look directly along the shaft of the tool with the eye contralateral to the tool projection (that is, using the eye on the same side as the cheek against which the tool is secured; Fig. 4b ), which is better positioned than the ipsilateral eye to maintain visual contact with the tool tip; meanwhile, the tool tip will lie closer to the central optical axis of the ipsilateral eye (that is, further from the limits of the retina). When the aperture of the hole was experimentally reduced in size, so that only one eye could see into the tube, our subjects proportionately increased the use of angled grips (for GLMM results, see above), which position both eyes equidistant to the line of the tool, bringing the eye that is ipsilateral during the angled grip closer to the tool ( Figs 3 and 4b ). In interspersed control trials, where the tube had a visual aperture large enough for both eyes to see into, but a small physical opening, our crows used an angled grip more frequently than a straight grip in comparison with the small aperture (GLMM: z =−2.99, P =0.003), although this was still a lower proportion of angled grips than that observed for the large aperture (GLMM: z =−4.37, P <0.001). This shows that the visual properties of a hole alone are sufficient to determine the tool grip used by NC crows while probing. 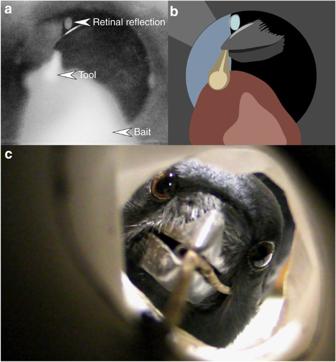Figure 3: Filming eye movements and tool-positioning in free-moving NC crows. (a) Single frame, shot with an infrared ophthalmoscope video camera, showing a crow using an angled tool grip, and (b) its schematic interpretation. The retinal reflection shows that the visual field of the contralateral eye embraces the tool-projection angle and that vision is not obstructed by the bill. The figure also shows that, in this instance, the ipsilateral eye cannot see the tool tip, highlighting the trade-off between various eye positions; whereas our behavioural experiments (see main text) indicate that the ipsilateral eye may be used preferentially (perhaps due to optical quality gains), the contralateral eye is able to provide more consistent coverage. The tube has a 35-mm diameter, which is considerably larger than most natural hole apertures19, but small enough to prevent the entire head from entering the tube. (c) Still image of a NC crow probing into a tube using a straight grip (note that the stick tool used in this pilot test was bent, whilst the tools used during experiments were straight), with both eyes rotated forward, clearly looking down the tool shaft. Figure 3: Filming eye movements and tool-positioning in free-moving NC crows. ( a ) Single frame, shot with an infrared ophthalmoscope video camera, showing a crow using an angled tool grip, and ( b ) its schematic interpretation. The retinal reflection shows that the visual field of the contralateral eye embraces the tool-projection angle and that vision is not obstructed by the bill. The figure also shows that, in this instance, the ipsilateral eye cannot see the tool tip, highlighting the trade-off between various eye positions; whereas our behavioural experiments (see main text) indicate that the ipsilateral eye may be used preferentially (perhaps due to optical quality gains), the contralateral eye is able to provide more consistent coverage. The tube has a 35-mm diameter, which is considerably larger than most natural hole apertures [19] , but small enough to prevent the entire head from entering the tube. ( c ) Still image of a NC crow probing into a tube using a straight grip (note that the stick tool used in this pilot test was bent, whilst the tools used during experiments were straight), with both eyes rotated forward, clearly looking down the tool shaft. 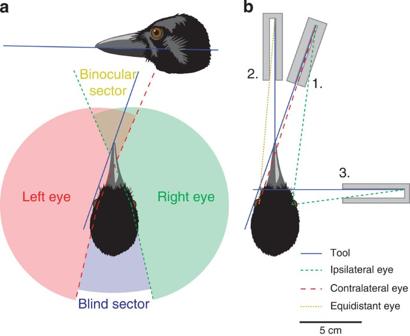Figure 4: Geometry of tool-holding in NC crows. (a) NC crows often hold tools using the tip of their bill, with the non-working end resting against the cheek, which presumably provides lateral stability9,10. This grip brings the tool into the NC crow's binocular sector where both eyes can see its working tip. (b) Illustration of the main grip modes that crows could theoretically use for extractive tool use. Holding the tool perpendicular to the bill (position 3) brings the tool tip into the field of the ipsilateral eye (green lines). The straight grip (position 2) allows either or both eyes to look along the tool. An angled grip (position 1) brings the tool into the field of the contralateral eye (red lines), allowing the contralateral eye to see into far smaller apertures than the ipsilateral eye. Owing to these geometric constraints, the hole aperture required for a clear view when holding the tool perpendicular to the bill (position 3) is approximately five times greater than that required in the angled grip position (position 1). Full size image Figure 4: Geometry of tool-holding in NC crows. ( a ) NC crows often hold tools using the tip of their bill, with the non-working end resting against the cheek, which presumably provides lateral stability [9] , [10] . This grip brings the tool into the NC crow's binocular sector where both eyes can see its working tip. ( b ) Illustration of the main grip modes that crows could theoretically use for extractive tool use. Holding the tool perpendicular to the bill (position 3) brings the tool tip into the field of the ipsilateral eye (green lines). The straight grip (position 2) allows either or both eyes to look along the tool. An angled grip (position 1) brings the tool into the field of the contralateral eye (red lines), allowing the contralateral eye to see into far smaller apertures than the ipsilateral eye. Owing to these geometric constraints, the hole aperture required for a clear view when holding the tool perpendicular to the bill (position 3) is approximately five times greater than that required in the angled grip position (position 1). Full size image Taken together, our behavioural experiments suggest that, as visual hole apertures become smaller, NC crows shift their grip to bring the (formerly) ipsilateral eye closer to the tool, enabling it to maintain visual contact with the tool tip. Further behavioural testing would be necessary to establish whether NC crows are able to utilize their large binocular fields for stereoscopic depth perception, which may be useful for gauging distances during tool deployment [11] . Bill shape and tool-projection angles We next combined our visual-field data with morphometric measurements, to assess whether any of our non-tool-using Corvus study species could, theoretically, achieve levels of physical and visual tool control similar to those inferred for NC crows. Tools can be securely held in the bill in several ways ( Fig. 4b ). In addition to the two principal modes described above, crows could hold stick tools perpendicular to the bill axis (position 3 in Fig. 4b ), so that the working tip of the tool can be positioned in a region covered by the visual field of the respective ipsilateral eye. However, such a grip positions the line of the tool further from the eye than an angled, or straight, grip (positions 1 and 2 in Fig. 4b ), making this grip less suitable for foraging in small holes (in Fig. 4b , an angled grip allows visual feedback from a hole aperture approximately five times smaller than a perpendicular grip). Intermediate angles between perpendicular and angled grips rely on the ipsilateral eye, and would therefore require an even larger aperture than a perpendicular grip. We modelled possible tool-projection angles that achieved, simultaneously, a stable tool grip, and the most direct view along the tool shaft. Each species' sagittal tool-projection angle was calculated from the angle of the maxilla where it intersects the mandibula at the bill tip (angle α in Fig. 5 ). In NC crows, this angle brings the tool into an approximately horizontal position below the eye where the non-working end of the tool can rest against the cheek (see above), presumably improving lateral stability during tool use. The curved bill characteristic of non-tool-using corvids [12] , on the other hand, results in significantly lower-elevation tool-projection angles ( Table 1 ), which consequently raises the non-working end of the tool above the eye where it cannot be secured against the cheek. Tools held by NC crows are estimated to project 'above' the bill tip (note that, similar to visual-field parameters, sagittal tool-projection angles were measured against the line connecting the bill tip and eye, which provides an unambiguous reference; compare Figs 4a and 5 ), which is consistent with observations of natural tool-projection angles [5] , [9] , [10] . In contrast, tools held by all other investigated Corvus species would fall below the bill tip ( Fig. 1 ). 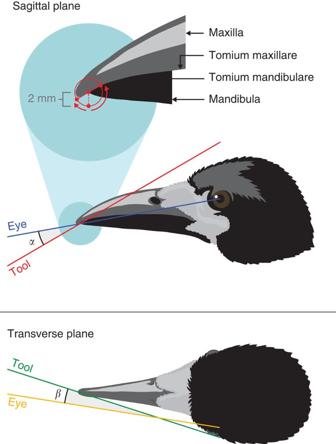Figure 5: Modelling of hypothetical tool-projection angles inCorvusspecies. The sagittal tool projection (angleα) is calculated from the angle of the maxilla's lower ridge where it intersects the mandibula (red) relative to a line from the bill tip to the eye (blue). The enlarged view of the bill tip shows how the tool-projection angle was estimated: assistants were asked to locate the point where the mandibula intersects the tomium maxillare, before rotating two radii around in each direction until the ends of the radii met the tomium maxillare (the average angle of these two radii was taken as the sagittal tool-projection angle). The transverse tool projection (angleβ) is calculated from the angle between the bill tip and a tangent to the outer edge of the eye (green) relative to the retinal field boundary at the elevation of the sagittal tool-projection angle (yellow). The figure shows the head of a rook as an example. Figure 5: Modelling of hypothetical tool-projection angles in Corvus species. The sagittal tool projection (angle α ) is calculated from the angle of the maxilla's lower ridge where it intersects the mandibula (red) relative to a line from the bill tip to the eye (blue). The enlarged view of the bill tip shows how the tool-projection angle was estimated: assistants were asked to locate the point where the mandibula intersects the tomium maxillare, before rotating two radii around in each direction until the ends of the radii met the tomium maxillare (the average angle of these two radii was taken as the sagittal tool-projection angle). The transverse tool projection (angle β ) is calculated from the angle between the bill tip and a tangent to the outer edge of the eye (green) relative to the retinal field boundary at the elevation of the sagittal tool-projection angle (yellow). The figure shows the head of a rook as an example. Full size image We also modelled transverse tool projections in each species when the tool is gripped in the bill tip at an angle as close to the eye as possible ( Figs 4 and 5 ), taking into account eye separation and bill length. Superimposing these tool projections on our estimated topographic maps of binocular fields revealed that, in contrast to results obtained for straight-billed NC crows, the curved maxilla of non-tool-using corvids forces the hypothetical tool into a position outside of their respective visual fields ( Fig. 1 and Table 1 ). Curved bills are thought to assist the visual inspection of the contents of the open bill in crow species probing in the ground or in carcasses [12] , [13] , suggesting that the NC crow has forgone this ability in favour of a bill shape that is suited to gripping and visually guiding tools. The rook C. frugilegus , a species that does not habitually use tools in the wild, has recently been shown to be a capable tool user in captivity [14] . Interestingly, our comparative results show that the rooks' ability to see along a tool is better than that of other non-tool-using crows, as a consequence of its moderate bill curvature (compare Figs 1 and 5 ). However, we note that the rooks used in earlier experiments [14] extracted bait from a transparent apparatus, so the limitations of their visual field could not be assessed. We suggest that future work further explores the envelope of conceivable tool grips, and resulting tool-projection angles, and cross-validates results with captive birds. We have presented a body of comparative data on the visual-field topography and bill morphology of six Corvus species, including: measurements from live, but restrained, birds; behavioural experiments with freely moving, naturally behaving NC crows; results from an exhaustive reanalysis of previously published data; and 3D topographical maps parameterized with measurements taken from live and museum specimens. Taken together, these multiple lines of investigation provide strong evidence that, perhaps uniquely among non-human animals [15] , [16] , NC crows possess morphological features that support tool-use behaviour. Although an earlier study had asserted that the visual-field topography of American crows may facilitate their 'rudimentary tool use' [8] , this claim is clearly unsupported by current evidence, as tool use has so far only been observed once in a single wild subject in this species [17] . In any case, the mean maximum binocular overlap of the American crow's visual field is much smaller than that observed in habitually tool-using NC crows, and falls well within the range of values obtained for the other non-tool-using Corvus species investigated in our study ( Fig. 2 , Table 1 ). It is currently impossible to establish causal relationships, because the number of tool-using bird species is insufficient for broad comparative analyses, and the current lack of NC crow (sub-)fossils prevents dating of key evolutionary events [6] . In other words, it remains an open question whether ancestors of NC crows possessed morphological features that predisposed them to tool manufacture and use, or whether tool-use behaviour was expressed first due to unusual ecological opportunities, before exerting selection pressures that gradually shaped the species' visual system and bill morphology [6] . Evidence that unusual ecological conditions have been major drivers in the evolution of habitual tool use is provided by detailed analysis of the foraging ecology of wild NC crows [6] , [18] , [19] and woodpecker finches Cactospiza pallida [20] , and the experimental results for rooks (see above). These avian study systems promise valuable, phylogenetically independent comparisons with the hominin lineage, where the evolution of opposable thumbs and flexible wrists in humans has enabled precision pinching and unprecedented tool-handling capabilities [2] , [3] , [4] , [15] , [16] , [21] . Visual-field measurements We used a well-established ophthalmoscopic reflex technique to measure visual-field parameters (monocular, binocular and cyclopean fields) and eye-movement amplitudes in 18 alert subjects across 6 Corvus species ( Table 1 ). This technique has been used in excess of 30 years on 46 bird species of different phylogeny, ecology and behaviour, permitting standardized interspecific comparisons [7] . The procedure is non-invasive and follows guidelines established by the United Kingdom's Animals (Scientific Procedures) Act (1986) and the Animal Welfare Act (2006). To locate subjects suitable for experimentation, we conducted an extensive search, using both our personal contacts and information found on the internet. We considered all species of the genus Corvus , and our final sample ( Table 1 ) reflects what could be achieved within the logistical constraints of our study. All experimental subjects were captive animals in the UK, Germany or Austria, with the exception of two ravens that were caught near the Konrad Lorenz Research Station in Grünau, Austria, as part of an ongoing field project. These two individuals were released back into the wild immediately after testing and marking. All other subjects were immediately returned to their home aviaries once measured. Each bird was held securely in a foam rubber cradle using fabric hook-and-loop fastener straps that wrap upon themselves ( Supplementary Fig. S1 ). The feet and legs were carefully tucked away beneath the bird, and the head was held in position with a bill-holder at the centre of a visual perimeter. To ensure a comfortable fit for the birds, we created species-specific bill-holders, using calibrated dorsal and lateral photographs of the heads of specimens from the Natural History Museum in Tring, UK (see below). Holders were made from aluminium and Polycaprolactone (thermoplastic, brand name: 'Polymorph') that could be moulded around the tip of the bill in situ . A fully adjustable, padded head-rest prevented the head from moving backwards, out of the holder. Each holder took account of the size and shape of the bill of the species being measured, and was further adjusted to fit individual subjects. The bill was held closed during experiments. Although subjects had to be restrained for 30–45 min, they could have been released from the apparatus immediately if they had shown any signs of distress (this was never necessary). For consistency, all visual-field measurements were made by the same experimenter (J.T.). The visual perimeter uses a conventional latitude and longitude system, with the equator aligned vertically at the angle between the eye and bill tip. The head is positioned so that the angle of the bill to the horizontal approximates that which the bird adopts spontaneously when held in the hand. Subjects' eyes were examined with an ophthalmoscope held against a perimeter arm, and longitudinal positions were recorded to ±1°. We established that the eyes of all subjects were mobile and could move independently. We determined the limits of the visual field, and the amplitude of eye movements, using the following procedure. The maximum and minimum longitudinal limits of the retinal visual field were measured in each eye at 10° (±1°) intervals of elevation (latitude). The limit of the visual field was determined by the projection of the limit of the retina, the ora serrata. This can be seen as a clear difference between the bright reflection from the retinal surface and the black of the ciliary folds. Because of eye movements, however, the visual projection of these limits is not fixed, so we recorded the maximum and minimum limits of the visual field at each elevation. These were defined by the positions that the retinal margins spontaneously adopted when the eyes were fully rotated 'forward' (converged) and 'backward' (diverged). To map these positions, successive measurements of the projection of the retinal margin at each elevation were made in quick succession, and the maximum and minimum values were recorded. The amplitude of eye movements at each elevation was taken as the difference between these maximum and minimum values. Eye movements are complex rotational movements, but our procedure enabled us to measure explicitly any consequent translational effects on the limits of the visual field at each elevation. At some elevations, eye movements made little discernible difference to the position of the field margins, whereas at other elevations, effects were more pronounced. Owing to inevitable obstruction by the holding apparatus, which varied in size across species (see above), visual-field parameters were measured down to different elevations in the lower part of the frontal field in different species ( Fig. 1 ). To the rear of the head, measurements were typically possible down to the horizontal plane. We also measured the optic axis of each eye (the line along which the cornea's and the lens' refractive surfaces are centred) by recording the perimeter coordinates at which the first and second Purkinje images (reflections from the cornea's and from the lens' anterior surface) of a point source of light held close to the line of sight were most closely aligned. To calculate the true angles of visual-field limits, rather than the angles observed from the perimeter arm of the apparatus, we had to account for the separation of each individual's eyes at the centre of the apparatus (320 mm from the perimeter arm). Angles measured from the perimeter arm were corrected from a hypothetical viewpoint to infinity from the nodal point of each eye [7] . Nodal separation was calculated from the distance between the cornea of each eye (measured from standardized and scaled digital photographs of the head of each subject held in the apparatus), and the divergence of the optic axes. This makes the assumption that the fundus (posterior portion of the eye) is semicircular and that the eyes meet in the sagittal plane of the skull. From these data we constructed a 3D topographical map of each species' visual fields, and assessed how field boundaries were affected by eye movements (see above). Importantly, our measurements for multiple subjects of the same species enabled us to compute species means and their associated s.e.m. for delineating field boundaries ( Fig. 1 ). This demonstrated that the degree of variation for boundaries was comparable across species, and that effect sizes in our comparisons of NC crows with the five other Corvus species substantially exceeded this intraspecific variation. The maximum width of the frontal binocular field (that is, maximum binocular overlap) was determined on the basis of mean values (see Table 1 ), to facilitate interspecific comparisons and functional interpretations based on the species' respective foraging ecologies. Collation of previously published visual-field data for reanalysis We attempted to collate all previously published data on the maximum binocular overlap in avian visual fields, using a research database that had been built up over the past 30 years (by G.R.M.) as well as systematic keyword searches ('bird* AND visual field*', 'bird* AND visual-field', 'avian AND visual field*' and 'avian AND visual-field*') in the 'Web of Knowledge' (Thompson Reuters) ( Supplementary Table S1 ; this search was completed on 15 April 2010). Measurement of hypothetical tool-projection angles We calculated the average sagittal tool-projection angle for each species from scaled macrophotographs taken of museum specimens (NC crow, n =3; carrion crow, n =5; jackdaw, n =3; raven, n =4; rook, n =3) and/or directly from the experimental subject where possible, that is, when the bill tip was not obscured by the bill holder (pied crow, n =1; rook, n =1). Although there are a number of conceivable ways in which a bird could hold a stick tool in its bill (three principal positions are schematically illustrated in Fig. 4b ), we chose to model an angled grip in the bill tip that would optimize the contralateral eye's alignment with the tool shaft (position 1 in Fig. 4b ) and presumably grant the greatest visual feedback during extractive tool use. Three assistants, who were blind with regards to the hypotheses under investigation, were independently shown a standardized and scaled photograph of each specimen on a computer screen, in a randomized order, and without reference to the species' identities. They were asked to locate the centre of the eye in each image and to position a circle, scaled to a 2-mm radius, where the tip of the mandibula intersects the tomium maxillare (the red circle in Fig. 5 ; for terminology, see Fig. 5 ). Next, they were asked to draw a radius from the centre of the bill-tip circle and rotate it clockwise from the 6-o'clock position until it touched the lowest point of the tomium, then repeat anti-clockwise. The average angle of the two radii was used to estimate sagittal tool-projection angles if each individual were to hold a tool in their bill tip (angle α in Fig. 5 ). Each experimental subject's mean transverse tool-projection angle was measured from the line between the bill tip and the outer edge of the centre of each eye relative to the left-right axis. The overlap between the transverse tool-projection angle and the limit of the subject's visual field at the elevation closest to the mean sagittal tool-projection angle of its species was then calculated (angle β in Fig. 5 ) to model each subject's ability to see parallel to the shaft of the tool. Behavioural experiments To film the eyes of unrestrained, naturally behaving NC crows during extractive foraging, we built a high-definition infrared ophthalmoscope from a commercial HD video camera (Sanyo Xacti HD2; 30 progressive frames per second; resolution 1280×780 pixels). The infrared-absorbing filter fitted to the camera's sensor was removed, and replaced with an infrared-transparent, visual spectrum-transparent filter made from acrylic. A film of reflective/transparent (50%/50%) mirror was used to align an infrared light-source with the camera's view, thus converting the system into an ophthalmoscope. Birds are not expected to be able to see the >750-nm wavelength output of the infrared ophthalmoscope, or through the opaque filter, which had a 720-nm cutoff [22] . Three wild-caught NC crows were housed temporarily in a field aviary (3×3×2 m) where they were given the opportunity to use supplied stick tools to extract beef-heart pieces from a horizontal tube, with the ophthalmoscope filming from the distal end ( Fig. 3 ). The first subject (A) was a female that was housed alone, and the two others (B and C) were a male and female of unknown relationship, housed with a juvenile they were feeding (but which did not participate in experiments). All three subjects had a dark-colour gape, suggesting they were adults [19] . The tube had a diameter of 35 mm, which was wide enough for crows to see the meat reward with both eyes simultaneously. Subjects were supplied with straight, 21 cm-long bamboo sticks, to standardize tool dimensions in experimental trials. Pieces of beef heart ( ca. 1 cm 3 ) were presented at a depth of 20 cm from the tube opening where they could not be reached by bill alone. Three experimental conditions were used: large aperture—the tube was left open so that both eyes could see the reward while probing (35-mm opening); small aperture—an opaque plate was fitted over the opening of the tube with a 20-mm diameter hole, preventing both eyes from seeing the reward simultaneously; and control—a transparent plate was fitted over the end of the tube with a 20-mm diameter hole to combine the physical obstruction of the small aperture, with the visual properties of the large aperture. As all plates were transparent to infrared, our ophthalmoscope could be used to film crow behaviour in all experimental conditions (that is, even through the opaque plate). We conducted a total of 118 trials across all subjects (crow A, n =80; crow B, n =10; crow C, n =28), with all three conditions presented in a semi-randomized order within birds. Both eyes were consistently in a forward position whenever they were visible across all subjects and trials. Grip type was categorized into right or left grip (tool projecting to the right or left of the bill), or central (tool projecting straight into the bill). Footage was scored in a frame-by-frame analysis by the same observer (J.T. ), noting each change of grip and duration of grip. A total of 747 tool grips were recorded (of which 479 were angled and 268 were straight). Crows exhibited clear laterality, holding the tool to one side of the head >99.9% of the time; crows A and B gripped the tools on their right sides, whereas crow C gripped the tool on its left side ( cf. [9] , [10] ). Average (±s.e.m.) grip duration was 3.4 s ±0.13. Statistical analyses Comparisons between Corvus species were conducted with general linear models, testing the null hypothesis that non-tool-using species do not differ from the NC crow in the chosen parameters (analyses excluded the pied crow and the American crow, because no replicate measurements were available for these species). Although sample sizes for general linear models were modest ( cf. Table 1 ), diagnostic scatter plots of standardized residuals, and post-hoc tests, indicated good model fit (normality of errors; homogeneity of variance). For illustration purposes (see Fig. 2 ), we constructed 95% confidence intervals for species means, using Student's t -distribution (rather than a normal distribution) because of small sample sizes [23] . No formal statistical comparisons were made with passerine and non-passerine species, because these are non-random samples that largely reflect research interests in the field of avian vision ecology over the past 30 years. It should be noted that our present analyses examine differences between species in absolute terms, but do not control for phylogenetic non-independence or other potentially confounding factors (such as body size). Although our work establishes beyond doubt that NC crows possess a highly unusual visual-field topography (for effect sizes, see main text, Fig. 2 and Table 1 ), both in comparison with congeneric and more distantly related species, formal phylogenetic analyses would be necessary to test more specific evolutionary hypotheses (for example, regarding the rates of evolutionary change in maximum binocular overlap). For analysing the results of our behavioural experiments, GLMMs were run in the lme4 package (0.999375-35), with a binomial error distribution (angled or straight tool grip) specified using the Laplace approximation. Experimental subject identity was included as a random effect on the intercept, and trial number was included as a random effect on the slope [23] . All statistical analyses were performed in R version 2.11.1 (ref. 24 ). How to cite this article : Troscianko, J. et al . Extreme binocular vision and a straight bill facilitate tool use in New Caledonian crows. Nat. Commun. 3:1110 doi: 10.1038/ncomms2111 (2012).